Current-induced self-switching of perpendicular magnetization in CoPt single layer All-electric switching of perpendicular magnetization is a prerequisite for the integration of fast, high-density, and low-power magnetic memories and magnetic logic devices into electric circuits. To date, the field-free spin-orbit torque (SOT) switching of perpendicular magnetization has been observed in SOT bilayer and trilayer systems through various asymmetric designs, which mainly aim to break the mirror symmetry. Here, we report that the perpendicular magnetization of Co x Pt 100- x single layers within a special composition range (20 < x < 56) can be deterministically switched by electrical current in the absence of external magnetic field. Specifically, the Co 30 Pt 70 shows the largest out-of-plane effective field efficiency and best switching performance. We demonstrate that this unique property arises from the cooperation of two structural mechanisms: the low crystal symmetry property at the Co platelet/Pt interfaces and the composition gradient along the thickness direction. Compared with that in bilayers or trilayers, the field-free switching in Co x Pt 100- x single layer greatly simplifies the SOT structure and avoids additional asymmetric designs. Current-induced spin-orbit torque (SOT) has been attracting great interest owing to its effective manipulation of magnetization [1] , [2] , [3] . The SOT switching of perpendicular magnetization usually requires extra assistance from external magnetic field in conventional heavy metal/ferromagnet (HM/FM) bilayers. To achieve the field-free switching, many efforts have been made to break the mirror symmetry relative to the xz plane, assuming the current is along the x direction and the magnetization is along the z direction [4] , [5] , [6] , [7] , [8] , [9] , [10] , [11] , [12] , [13] , [14] . It can be realized by introducing a tilting effect (such as tilted structure [4] , [5] or tilted anisotropy [6] , [7] ) in the yz plane, a polar vector (such as electrical field [8] or electric polarization) along the y direction, and an axis vector (such as interlayer coupling [9] , exchange bias [10] , [11] , [12] , stray field [13] , or additional magnetic layer [14] ) along the x direction. The chiral symmetry breaking by a gradient of magnetic anisotropy or saturation magnetization can also induce field-free switching [15] . Different from the above approaches that require asymmetric designs in device/film structures, recent works utilized the crystal symmetry to engineer the field-free switching in the WTe 2 /FM bilayer [16] , [17] , [18] and the CuPt/FM bilayer [19] . Although largely explored, the existing field-free switching in the above SOT bilayers/trilayers has some intrinsic disadvantages. First, the SOT (usually generated from an individual spin source layer) is an interface effect in nature, which constrains the thickness of the FM layer and limits the thermal stability of the memory cell. Second, the interfacial spin mixing may lead to a decrease in the switching efficiency. Therefore, it has been desirable to explore the current-induced field-free switching in a single ferromagnetic layer. Previously, current-induced perpendicular magnetization switching in the single magnetic layer by bulk SOT has been demonstrated in diluted ferromagnets (GaMnAs [20] , GeMnTe [21] ) with bulk inversion asymmetry, which however requires low temperature and external in-plane magnetic field. The SOT switching in a single layer of metallic ferromagnets ( L 1 0 -FePt [22] , [23] , CoTb [24] ) by composition gradient or inner interface-induced inversion asymmetry brings the working temperature to 300 K, though the external in-plane magnetic field is still needed. Recently, the field-free SOT switching is realized by gradient-driven Dzyaloshinskii–Moriya interaction (DMI) induced by composition gradient in a CoTb layer [25] , where the deterministic switching starts with the domain nucleation at the edge of the sample due to the magnetization tilting. Here we report on the observation of the current-induced field-free switching of perpendicular magnetization in Co x Pt 1- x single layers by combining the composition gradient-induced damping-like torque and the low crystal symmetry-induced “3m torque”. We show that the SOT in Co x Pt 1- x can be largely tuned by changing the composition ratio from x = 20 to x = 56, and the specific composition of Co 30 Pt 70 was found to exhibit the best SOT switching performance. Based on the thickness and the composition dependences, we suggested that the field-free SOT switching in Co 30 Pt 70 is closely related to the formation of Co platelets near the substrate. Structural and magnetic properties In general, the Co x Pt 1- x alloys have different phases with varied compositions, including the chemically ordered L 1 2 , L 1 0 , L 1 1 , and D 0 19 phases and the disordered A1 and A3 phases. Among all phases, the A1 disordered CoPt 3 (with a certain x range) possesses low saturation magnetization ( M s ), which is desirable for energy-efficient magnetization switching. In our experiments, we deposited Co 30 Pt 70 films with thicknesses varying from 6 to 12 nm on single-crystalline MgO (111) substrate at 300 °C (see the “Methods” section). The composition of Co 30 Pt 70 was verified by energy-dispersive X-ray spectroscopy (EDS). It has been reported that the A1 disordered CoPt 3 with a face-centered cubic ( fcc ) structure has perpendicular magnetic anisotropy (PMA) due to the excess of the in-plane Co–Co bonds with the formation of Co platelets on Pt-rich matrix during growth [26] , [27] , [28] , [29] . To confirm the bonding anisotropy in our Co 30 Pt 70 films, we performed the X-ray absorption spectroscopy (XAFS) experiments and Supplementary Table S1 summarized the fitted parameters for different bonds in the in-plane directions and the out-of-plane directions (Supplementary Section 1). We found a dominated Co–Co in-plane pairing, which indicates the formation of Co platelets. The structure of Co 30 Pt 70 with Co platelets is schematically illustrated on the left of Fig. 1a . The right top of Fig. 1a shows a side view of the Co platelet/Pt, which resembles the Co/Pt superlattice. The right bottom of Fig. 1a shows the top view of the Co platelet/Pt structure, where the in-plane mirror symmetry is broken with respect to the (11-2) plane (defined by [1-10] and [111]), while preserved with respect to the (1-10) plane (defined by [11-2] and [111]). According to the previous studies, the broken in-plane mirror symmetry would allow for an out-of-plane (OOP) spin-orbit torque [16] . The high-resolution transmission electron microscopy (HR-TEM) result of our Co 30 Pt 70 in Fig. 1b shows a stacking sequence of ABCABC… from bottom to top, which is consistent with its fcc structure (see Supplementary Section 1 for more discussions). 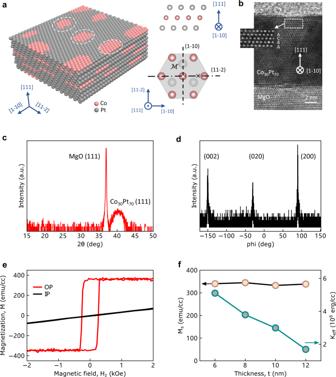Fig. 1: Structural and magnetic properties of Co30Pt70thin film. aLeft: the schematic illustration of Co30Pt70with randomly located Co platelets (see white circles); right top: the side view of the Co platelet/Pt structure; right bottom, the mirror symmetry analysis of Co platelet/Pt, where [1-10] is defined as the low-symmetry axis and [11-2] as the high-symmetry axis, respectively.bHigh-resolution transmission electron microscopy (HR-TEM) image of Co30Pt70with [1-10] pointing inward. The area within the dotted rectangle was amplified to present the stacking sequence (ABCABC…, from bottom to top) of Co30Pt70.cHigh-resolution X-ray diffraction (HR-XRD) pattern of Co30Pt70.dHR-XRD phi-scan pattern with Co30Pt70(002) plane rotated along [111] axis.eOut-of-plane (OP) and in-plane (IP) magnetic hysteresis loops of the unpatterned Co30Pt70thin film.fThickness dependence of the saturation magnetization (Ms) and effective perpendicular magnetic anisotropy energy (Keff). Figure 1c shows the high-resolution X-ray diffraction (HR-XRD) pattern of a 6 nm Co 30 Pt 70 thin film with a (111) peak at 40.6°. The phi-scan pattern in Fig. 1d shows three peaks that indicate the three-fold rotational symmetry. The TEM and XRD results verified the fcc structure and the epitaxial growth of our Co 30 Pt 70 film. Figure 1e shows the magnetic hysteresis ( M-H ) loops of the 6 nm Co 30 Pt 70 thin film, where the squared out-of-plane M-H loop and the linear in-plane M-H relation indicate a good PMA. The M - H loops for Co 30 Pt 70 with various thicknesses from 6 to 12 nm are shown in Supplementary Fig. S2 . As summarized in Fig. 1f , the saturation magnetization ( M s ) remains almost constant with changing thickness, while the effective perpendicular magnetic anisotropy energy ( K eff ) shows a decreasing trend with thickness, indicating that the Co platelets mainly exist near the substrate. Fig. 1: Structural and magnetic properties of Co 30 Pt 70 thin film. a Left: the schematic illustration of Co 30 Pt 70 with randomly located Co platelets (see white circles); right top: the side view of the Co platelet/Pt structure; right bottom, the mirror symmetry analysis of Co platelet/Pt, where [1-10] is defined as the low-symmetry axis and [11-2] as the high-symmetry axis, respectively. b High-resolution transmission electron microscopy (HR-TEM) image of Co 30 Pt 70 with [1-10] pointing inward. The area within the dotted rectangle was amplified to present the stacking sequence (ABCABC…, from bottom to top) of Co 30 Pt 70 . c High-resolution X-ray diffraction (HR-XRD) pattern of Co 30 Pt 70 . d HR-XRD phi-scan pattern with Co 30 Pt 70 (002) plane rotated along [111] axis. e Out-of-plane (OP) and in-plane (IP) magnetic hysteresis loops of the unpatterned Co 30 Pt 70 thin film. f Thickness dependence of the saturation magnetization ( M s ) and effective perpendicular magnetic anisotropy energy ( K eff ). Full size image Current-induced SOT effective fields and field-free switching We patterned the Co 30 Pt 70 film into Hall bar devices for electrical transport measurements (see “Methods”). We changed the current angle θ I relative to the [1-10] crystal axis to investigate the crystal symmetry-dependent properties, as illustrated in Fig. 2a . θ I = 0, 60, 120, 180° and θ I = 30, 90, 150° represent that the current is applied along the low-symmetry axes and high-symmetry axes, respectively. 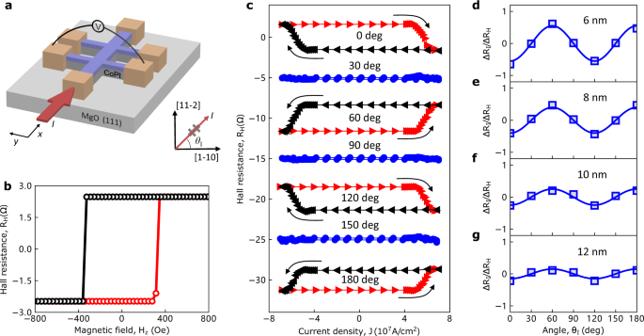Fig. 2: Field-free magnetization switching in Co30Pt70single layers on MgO (111) substrate. aSchematic of the Co30Pt70Hall bar device for electrical transport measurement.bAnomalous Hall effect of the 6 nm Co30Pt70sample.cCurrent-induced field-free magnetization switching in Co30Pt70for Hall bars with differentθI. The loops are manually shifted for better visualization.d–gθIdependence of ΔRI/ΔRHfor Co30Pt70devices with different thicknesses (6, 8, 10, and 12 nm). Figure 2b shows the anomalous Hall loop of the 6 nm Co 30 Pt 70 device, which agrees with its good PMA. The current-induced field-free magnetization switching loops for varying θ I are shown in Fig. 2c . We found that there is no obvious switching loop when the current is applied along the high-symmetry axes. In contrast, the switching loops appeared when the current is applied along the low-symmetry axes. In addition, the switching loop polarities for two adjacent low-symmetry axes (for example 0 and 60°) are opposite. The switched resistance Δ R I is defined to be the difference between the Hall resistance when the current pulse is swept from positive maximum to 0 mA and that when the current pulse is swept from negative maximum to 0 mA. Figure 2d shows the θ I dependence of the switching ratio Δ R I /Δ R H of the 6 nm sample, where Δ R H is the Hall resistance change in the AHE loop. The 120° periodic switching behavior is consistent with the three-fold in-plane rotational symmetry of Co platelet/Pt at the interface. This three-fold angular-dependence of the field-free magnetization switching also exists in Co 30 Pt 70 devices with varied thicknesses from 8 to 12 nm (Fig. 2e–g ), whose anomalous Hall loops and current-induced magnetization switching loops for different θ I values are shown in Supplementary Fig. S4 and S5 , respectively. We found that Δ R I /Δ R H decreases with the increasing thickness (Supplementary Fig. S6 ), which could be explained if the Co platelets mainly exist near the substrate. Fig. 2: Field-free magnetization switching in Co 30 Pt 70 single layers on MgO (111) substrate. a Schematic of the Co 30 Pt 70 Hall bar device for electrical transport measurement. b Anomalous Hall effect of the 6 nm Co 30 Pt 70 sample. c Current-induced field-free magnetization switching in Co 30 Pt 70 for Hall bars with different θ I . The loops are manually shifted for better visualization. d – g θ I dependence of Δ R I /Δ R H for Co 30 Pt 70 devices with different thicknesses (6, 8, 10, and 12 nm). Full size image To reveal the origin of the current-driven switching, we first characterized the out-of-plane effective field (Δ H OOP ) of the devices by measuring the anomalous Hall loops under positive and negative pulsed d.c . currents for different θ I , as shown in Fig. 3a, b and Supplementary Figs. S7 . 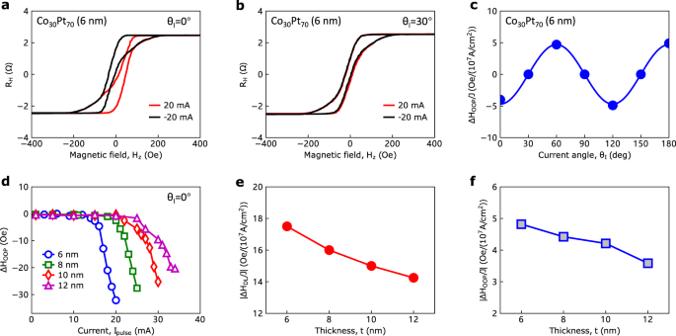Fig. 3: Current-induced out-of-plane and in-plane SOT effective fields. a,bAHE loops under +20 and −20 mA pulsed currents forθI= 0° (a) and 30° (b).cCurrent angle dependence of the out-of-plane effective field efficiency (ΔHOOP/J) in 6 nm Co30Pt70.dCurrent dependence of ΔHOOPfor various Co30Pt70thicknesses.e,fThickness dependences of in-plane and out-of-plane SOT effective fields forθI= 0°, respectively. The ΔHOOPfor the largest measured current in (d) is used for the calculation in (f). Figure 3c shows the θ I dependent out-of-plane effective field efficiency (Δ H OOP / J ), by using the Δ H OOP measured at 20 mA. The three-fold angular-dependent property is in accordance with that for the current-induced field-free switching. The current dependences of Δ H OOP / J for different Co 30 Pt 70 thicknesses are shown in Fig. 3d , where we observed different current thresholds above which the Δ H OOP / J values start to emerge and grow rapidly (Supplementary Section 4). We also estimated the in-plane damping-like effective field by harmonic Hall measurements (see Supplementary Sections 5 and 6). Figure 3e and f show that both the in-plane damping-like effective field efficiency (Δ H DL / J ) and Δ H OOP / J decrease slowly with increasing thickness. Then we measured the Δ H DL and the DMI field ( H DMI ) for varying θ I in our Co 30 Pt 70 single layer (see Supplementary Section 7). We found that both H DMI and Δ H DL are isotropic with θ I (Supplementary Fig. S17 ), in contrast to the anisotropic behavior of Δ H OOP . Next, we studied the reversal mode [30] of the magnetization during the SOT switching. We performed microscopy imaging of the magneto-optical Kerr effect (MOKE) on the device, as shown in Supplementary Section 8. By comparing the experiments with and without external magnetic field, we found that the reversal mode of the field-free switching in our Co 30 Pt 70 single layer is dominated by domain nucleation. We note that the behavior and the origin of the field-free switching in Co 30 Pt 70 are quite different from that recently reported in the CoTb layer [25] . First, the field-free switching in ref. [25] starts with the nucleation of a domain at the edge of the sample due to the gradient DMI. While the field-free switching of Co 30 Pt 70 starts with the nucleation of the domains mostly at the center part of the bar device, where the current density is the largest. Second, the antisymmetric DMI-induced field-free switching should have a one-fold angular dependence (with a period of 360°) on the in-plane current angle ( θ I ). In contrast, the field-free SOT switching in Co 30 Pt 70 shows a three-fold angular dependence on θ I . Therefore, the crystal symmetry, instead of the DMI, plays a key role in the three-fold field-free switching in Co 30 Pt 70 . Furthermore, the M-H curves under different in-plane magnetic field directions (Supplementary Fig. S3 ) do not show any noticeable anisotropy, which rules out the effect of the magnetic easy axis tilting on the free field switching. To study if the change of the substrate can influence the switching behavior or not, we prepared a 6 nm Co 30 Pt 70 sample on SrTiO 3 (111) substrate. We found that the switching behavior (Supplementary Fig. S22c ) for Co 30 Pt 70 /SrTiO 3 (111) is almost the same as that (Fig. 2c ) for Co 30 Pt 70 /MgO (111), which excludes the influence of substrate change and suggests a self-switching characteristic in the Co 30 Pt 70 layer. Fig. 3: Current-induced out-of-plane and in-plane SOT effective fields. a , b AHE loops under +20 and −20 mA pulsed currents for θ I = 0° ( a ) and 30° ( b ). c Current angle dependence of the out-of-plane effective field efficiency (Δ H OOP / J ) in 6 nm Co 30 Pt 70. d Current dependence of Δ H OOP for various Co 30 Pt 70 thicknesses. e , f Thickness dependences of in-plane and out-of-plane SOT effective fields for θ I = 0°, respectively. The Δ H OOP for the largest measured current in ( d ) is used for the calculation in ( f ). Full size image Composition dependence of the switching performance For further study, we investigated the field-free switching behavior in 6 nm Co x Pt 100- x on SrTiO 3 (111) with x ranging from 20 to 56. The magnetic and structural properties for these Co x Pt 1- x samples are shown in Supplementary Fig. S20 and S21 , all showing good PMA and good epitaxial growth. Their XRD results are better than that of Co 30 Pt 70 /MgO (111). In Fig. 4d , the saturation magnetization M s and the effective perpendicular anisotropy energy K eff increase with increasing Co composition from 20% to 56%, consistent with previous reports [31] , [32] , [33] . We performed the current-induced magnetization switching and OOP effective field measurements for these Co x Pt 100- x samples, as shown in Supplementary Fig. S22 and S24 . We found that Co 30 Pt 70 shows the most prominent switching behavior with the highest Δ R I /Δ R H ratio, as summarized in Fig. 4e . With x decreasing or increasing from 30, the field-free switching ratio decreases. 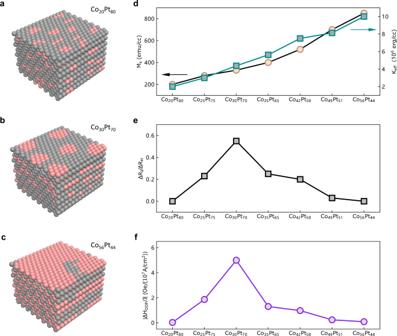Fig. 4: Composition dependence of the OOP effective fields and switching behavior in CoxPt100-xsingle layers on SrTiO3(111) substrates. a–cTentative structures of Co20Pt80, Co30Pt70, and Co56Pt44, which correspond to the lowest, optimal and highest Co compositions in our experiments, respectively. A large disordered background was omitted in these structures for easier analysis. Since the Co platelets are mainly distributed near the substrate, the top side of the structure in (b) is adjacent to the substrate.dComposition dependence ofMsandKeffin CoxPt100-xsingle layers.eComposition dependence of ΔRI/ ΔRHin CoxPt100-xsingle layers.fComposition dependence of ΔHOOP/Jin CoxPt100-xsingle layers. Figure 4f shows that the largest Δ H OOP / J also appears in Co 30 Pt 70 , following the behavior of Δ R I /Δ R H . To interpret the above phenomena, we tentatively make a comparison among three typical compositions (Co 20 Pt 80 , Co 30 Pt 70 , and Co 56 Pt 44 ), whose structures are schematically shown in Fig. 4a–c , respectively. For Co 20 Pt 80 , we assume that the Co clusters are small and randomly distributed in the Pt matrix, as shown in Fig. 4a . For Co 56 Pt 44 in Fig. 4c , alternative stacking of Co and Pt in long-range order can be formed, giving rise to an L 1 1 ordered CoPt under certain growth conditions. We note that the nominal chemical ordering parameter ( S ) for the presented Co 56 Pt 44 structure in Fig. 4c is close to 1. However, in experiments, the S value is usually lower than 0.3 because the L 1 1 CoPt is a metastable phase. Therefore, a large portion of the structure should be occupied by a randomly distributed Co and Pt (almost fully disordered) background. Similar disordered backgrounds may also exist in Co 20 Pt 80 and Co 30 Pt 70 . However, since a fully disordered background will not allow for the OOP SOT by symmetry, we ignore its existence in Fig. 4a–c for simplicity. Then we can make the symmetry analysis of the three typical structures. For Co 20 Pt 80 , the small composition ratio of Co makes it difficult to form large Co platelets, and the OOP SOT is unlikely to generate in those randomly distributed small Co clusters. For Co 56 Pt 44 , the long-range atomically ordered [Co/Pt] N is close to L 1 1 CoPt, which adopts the point group \(R\bar{3}m\) in the bulk. It is only at the substrate/film interface that the point group can reduce to 3m1, which gives rise to a finite 3m torque [19] . In addition, the large saturation magnetization and anisotropy energy in Co 56 Pt 44 (Fig. 4d ) also make it more difficult to be switched compared with the other compositions. For Co 30 Pt 70 , the Co platelets are not enough to form a long-range atomically ordered [Co/Pt] N structure, but can create a relatively large portion of Co platelet/Pt structures. More importantly, the Co platelets mainly distribute within several nanometers near the substrate. It is likely that the numbers of the Co platelets show a decreasing trend from the bottom (near the substrate) to the top (near the surface). This could be the reason why we can have a sizable 3m torque in our Co 30 Pt 70 sample. Fig. 4: Composition dependence of the OOP effective fields and switching behavior in Co x Pt 100- x single layers on SrTiO 3 (111) substrates. a – c Tentative structures of Co 20 Pt 80 , Co 30 Pt 70 , and Co 56 Pt 44 , which correspond to the lowest, optimal and highest Co compositions in our experiments, respectively. A large disordered background was omitted in these structures for easier analysis. Since the Co platelets are mainly distributed near the substrate, the top side of the structure in ( b ) is adjacent to the substrate. d Composition dependence of M s and K eff in Co x Pt 100-x single layers. e Composition dependence of Δ R I / Δ R H in Co x Pt 100-x single layers. f Composition dependence of Δ H OOP / J in Co x Pt 100-x single layers. Full size image Origin of the damping-like spin-orbit torque Next, we explored the origin of in-plane damping-like torque in the Co 30 Pt 70 single layer. Previously, the L 1 0 FePt single layer has been reported to exhibit current-induced bulk SOT due to the composition gradient along the thickness direction [22] , [23] . The bulk SOT has also been reported to exist in CoTb [24] , [34] , GdFeCo [35] , disordered-CoPt [36] , and disordered-Fe x Pt 1- x [37] single layers. We checked the composition distributions of Co and Pt in the 12 and 6 nm Co 30 Pt 70 film along the film thickness direction by using high-angle annular dark-field scanning transmission electron microscopy (HADDF-STEM), as shown in Supplementary Fig. S25 . We found that the Co/Pt ratio for the 12 nm film changes from 30:70 at the bottom of the film to 27:73 at the top and the composition gradient is estimated to be 0.5%/nm by a linear fitting. The composition gradient of the 6 nm Co 30 Pt 70 is 1.85%/nm, which is larger than that of the 12 nm Co 30 Pt 70 . This could be one of the reasons why the damping-like effective field of 6 nm is larger than that in 12 nm Co 30 Pt 70 (Fig. 3e ). To further verify if the composition gradient in the Co 30 Pt 70 single layer plays the main role in generating the damping-like effective field or not, we fabricated two control samples with designed positive and negative composition gradients along the film’s normal direction. Then we conducted the current-induced switching experiments and found that the switching polarity reverses when the composition gradient is reversed (Supplementary Fig. S26 ). Because the current-induced magnetization switching under assistant in-plane magnetic field is mainly driven by the damping-like SOT, the reversal of the switching polarity indicates a sign change in the damping-like SOT. Therefore, we concluded that the damping-like SOT in Co 30 Pt 70 should mainly come from the composition gradient. If we compare the switching loops of Co 30 Pt 70 (in Fig. 2c ) and that of CuPt/CoPt in our previous work [19] , we found their switching polarities are opposite. For example, when θ I = 0°, the switching polarity is clockwise for Co 30 Pt 70 while anti-clockwise for CuPt/CoPt. Based on our 3m torque model [19] , the sign of the 3m torque (along + z or − z ) is determined by the sign of the damping-like torque. Therefore, the opposite switching polarities for the two systems mean that their damping-like torques have opposite signs. This could be due to the fact that the CuPt spin source layer locates at the bottom of CoPt for the CuPt/CoPt bilayer, while for the Co 30 Pt 70 single layer, there is Pt segregation on the top side of the layer. In order to test the robustness of the field-free switching in Co 30 Pt 70 , we performed a switching cycling test by applying positive and negative pulsed currents repeatedly. After 15,000 circles, we observed that Δ R I almost keeps unchanged (Supplementary Fig. S27 ), which indicates a good endurance. We note that the switching ratio for our Co 30 Pt 70 doesn’t exceed 60%, which could be mainly due to the pinning effect from the magnetic Hall arms. Since it is not possible to make a pillar structure [19] in the single-layer form, we suggest one can use non-magnetic Hall voltage arms (such as Ti/Cu electrodes) to avoid the pinning effect and improve the switching ratio [38] . In summary, we report the observation of the current-induced field-free switching in Co x Pt 100- x single layers. By studying the SOT in Co x Pt 100- x with varying x from 20 to 56, we found that the Co 30 Pt 70 has the largest OOP effective field efficiency and best field-free switching performance. The origin of the field-free switching in Co 30 Pt 70 is attributed to the formation of Co platelets and the composition gradient in the film’s normal direction. The composition gradient along film normal direction gives rise to the in-plane damping-like torque while the low symmetry (3m1) property at the interface of Co platelet/Pt gives rise to the 3m torque. The cooperation of these two effects leads to a three-fold field-free switching in the Co 30 Pt 70 single layer. Our result of the self-switching in Co 30 Pt 70 has provided one of the most simplified structures for field-free switching of perpendicular magnetization. The good endurance and high thermal stability make it a good candidate for magnetic memory devices and other spintronic applications. Our work may stimulate further investigation of the current-induced self-switching in single-layer systems. Sample growth and device fabrication Co x Pt 100- x single layers were epitaxially deposited on MgO (111) and SrTiO 3 (111) single-crystal substrate by d.c . magnetron sputtering (AJA). The base pressures were lower than 4 × 10 −8 Torr. The Ar gas pressure was kept a constant at 5 mTorr. The temperature was kept at 300 °C during the deposition process, then the film was left to cool down to room temperature and a 2 nm SiO 2 protection layer was deposited as protection. After deposition, the films were patterned into 5 μm Hall bars with different in-plane orientations by using laser writer and Ar ion milling. Then the contact electrode pattern was defined by laser writer, followed by the deposition of Ti (7 nm)/Cu (100 nm) and the lift-off process. Current-induced switching measurement For the current-induced magnetization switching measurement, a pulsed d.c . electrical current with a duration of 30 μs was applied. After 8 s, the Hall resistance was recorded by using a small a.c . excitation current (50 μA). Current-induced out-of-plane effective field measurement For each data point in the AHE loop when measuring the out-of-plane effective field, we first swept the external out-of-plane magnetic field to a target value (such as H z = 20 Oe), then we applied a current pulse (such as I pulse = 18 mA) with a pulse width of 30 μs. After 6 s of the applied pulsed current, we applied a small ac current to detect the Hall resistance. TEM sample preparation and characterization TEM samples of the Co 30 Pt 70 single layer were fabricated by a focused ion beam machine (FEI Versa 3D system). The sample was thinned down using a Ga ion beam first with an accelerating voltage of 30 kV and then 8 kV. After that, the sample was polished by a 2 kV ion beam. Microstructures were studied by transmission electron microscopy (TEM) (JEOL JEM-2100F) at an accelerating voltage of 200 kV with energy-dispersive X-ray spectroscopy (EDS) analysis performed in scanning transmission electron microscopy (STEM) mode.